Developmental correspondence between action prediction and motor ability in early infancy How do infants understand the goals of others' actions? It has been proposed that action-understanding results from a mechanism whereby an observed action is mapped onto the observer's own motor representation of that action. However, direct evidence of the matching process in early infancy is difficult to find. Here we show the developmental correspondence between action prediction and motor ability by comparing gazing and grasping responses to interesting objects in 4- to 10-month-old infants and adults. The onset of infants' ability to predict the goal of others' action was found to be synchronized with the onset of their own ability to perform that action. Moreover, there was correspondence relationship between action-prediction ability and motor ability of same action. Our findings indicate that the ability to predict others' action goals requires a corresponding motor ability, providing ontogenetic evidence for a direct matching process by a mirror neuron system. How do infants understand the goals of others' actions? Neurophysiological [1] , [2] , [3] , [4] , [5] , [6] , [7] and brain-imaging [8] , [9] , [10] , [11] studies indicate that others' actions are understood through a direct matching process of a mirror neuron system (MNS), where an observed action is mapped onto the observer's own motor representation of that action [12] , [13] . In fact, several recent neurophysiological studies with infants over the age of 6 months have shown MNS functioning when the infants observed others' actions [14] , [15] , [16] , [17] , [18] , [19] . In spite of this correlation, compelling evidence of the direct matching process in early infancy is rare. Recent neurophysiological studies found that motor activation in areas associated with the MNS occurred immediately prior to the onset of observed actions in adults [20] and 9-month-olds [17] . Moreover, recent behavioural studies showed that adults [21] and 12-month-old infants [22] manifest proactive goal-directed eye movements while observing the manipulating actions of others. Taken together, developmental eye movement and neurophysiological studies suggest a promising avenue for research to elucidate the ontogenetic mechanisms of the direct matching process in the MNS. According to the direct matching hypothesis [12] , [13] , understanding of the actions of others derives from translating them into the repertoire of the observer's own actions. Theoretically, this implies that actions of others are only understood when an observed action is within the observer's motor repertoire. If a direct matching process in the MNS mediates the ability to predict an action, then there should be synchrony in the developmental trajectory between the onset of ability to predict others' action goals and the onset of infants' ability to perform that action. Moreover, the direct matching hypothesis also implies that the matching process requires a systematic correspondence between visual activity involved in observing actions and the actions available in the observer's motor repertoire. Thus, the relationship between the ability to predict others' action goals and one's own ability to perform that action should have a correspondence. The ontogeny of the direct matching process of the MNS has been a focus of much research [23] , [24] . In fact, some developmental studies have demonstrated that the perception of actions and their execution have mutual influence [25] , [26] , [27] , and that there exists an association between action perception and action execution [28] . However, to date, no studies have investigated the possibility of a correspondence relationship between the development of action understanding and the development of motor ability for performing the same action in early infancy. Addressing this issue can provide converging evidence regarding the development of the direct matching process predicted by the MNS. Here we report evidence to suggest that the developmental onset of infants' ability to understand an action, reflected by the ability to predict the goal of others' action, is synchronized with the developmental onset of their own ability to perform that action, and that there is developmental correspondence relationship between the ability to predict the goal of an action and the ability to perform that same motor action. From early infancy (around 6 months), grasping responses have been interpreted as goal-directed [29] , and are actions within the range of those possible at this stage of life [30] , [31] . Furthermore, many developmental studies that have relied upon grasping responses have used various groups of infants with ages less than 9 months [15] , [17] , [18] , [19] , [32] . Accordingly, we used grasping as a type of action for which young infants are likely to have a motor representation and are capable of performing. In this study, we investigated the developmental correspondence between action prediction and motor ability by comparing gazing and grasping responses to interesting objects in 4-, 6-, 8-, and 10-month-old infants and adults. We found that the onset of infants' ability to predict the goal of others' grasping action was synchronized with the onset of their own ability to perform that action. In addition, there was correspondence relationship between the action prediction ability and motor ability of same action. These findings indicate that the ability to predict others' action goals requires a corresponding motor ability. Our findings provide direct ontogenetic evidence for a direct matching process by a MNS. To investigate developmental correspondence between the ability to predict others' action goal and motor ability to perform this action, we presented action prediction task and grasping task to the infants, and compared their eye-movement responses with those of adults. In action prediction task, the videos showed three types of actions: 'grasping hand' (goal-directed action; GH condition), 'back of hand' (non-goal-directed or non-purposeful action [33] , BH condition), and 'mechanical claw' (inanimate goal-directed action; MC condition). In principle, the MNS should not be activated by either non-goal-directed [34] , [35] or inanimate actions [36] , [37] (BH and MC conditions). In addition, neither of the actions in the conditions corresponded systematically to actions identified within the motor repertoire of these infants. Thus, we expected that infants would not predict the action goals of others in BH and MC conditions even if infants were able to grasp. The Methods section, Fig. 1 , and Supplementary Movies 1-3 provide more complete details of these actions and conditions. Using an eye-tracking technique, we measured the time of the gaze arrival at the goal relative to the arrival of the observed agents' actions as an index of action prediction ability (Methods and Fig. 2a ). 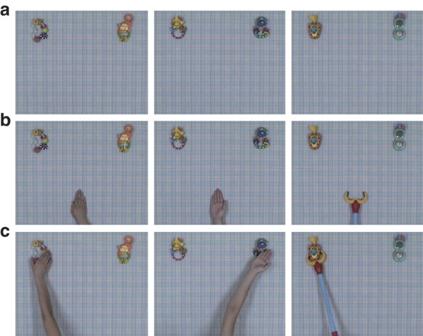Figure 1: Selected frames from the video stimuli of each condition. Each condition is grasping hand (GH, left panels), back of hand (BH, middle panels), and mechanical claw (MC, right panels) condition. (a) The agents are out of frame. (b) The agents appear from the bottom of the frame and move upward, and then stop. (c) The agents move towards one of two toys, stop at the target toy, and then make contact by grasping (GH, MC) or touching with back of hand (BH). Figure 1: Selected frames from the video stimuli of each condition. Each condition is grasping hand (GH, left panels), back of hand (BH, middle panels), and mechanical claw (MC, right panels) condition. ( a ) The agents are out of frame. ( b ) The agents appear from the bottom of the frame and move upward, and then stop. ( c ) The agents move towards one of two toys, stop at the target toy, and then make contact by grasping (GH, MC) or touching with back of hand (BH). 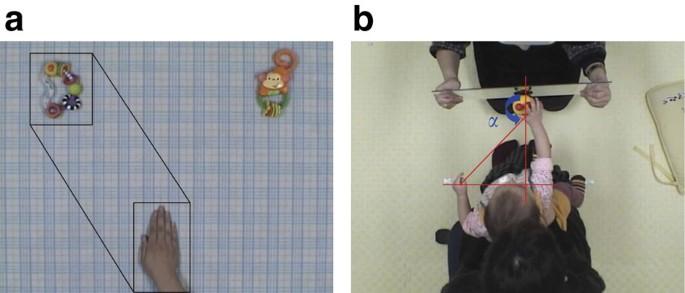Figure 2: Analytical examples of stimulus video and grasping ability. (a) Example of the video of grasping hand condition. Black rectangles and hexagon represent AOIs within the scene. The upper AOI was labelled 'goal AOI', encompassing the target object. The lower AOI was labelled 'agent AOI', encompassing the position in which agent stopped before the agent began to move to the target object. The middle AOI was labelled 'trajectory AOI', encompassing the trajectory of the agent's movement. (b) Example of grasping ability analysis. The geometry used to calculate the relative alignment of the infant's grasping action. The angle α was calculated for each analysed frame of the infant's contact with the object display. An α angle value from 90 to 180° indicates that the infant is engaged in a one-handed grasping action. Full size image Figure 2: Analytical examples of stimulus video and grasping ability. ( a ) Example of the video of grasping hand condition. Black rectangles and hexagon represent AOIs within the scene. The upper AOI was labelled 'goal AOI', encompassing the target object. The lower AOI was labelled 'agent AOI', encompassing the position in which agent stopped before the agent began to move to the target object. The middle AOI was labelled 'trajectory AOI', encompassing the trajectory of the agent's movement. ( b ) Example of grasping ability analysis. The geometry used to calculate the relative alignment of the infant's grasping action. The angle α was calculated for each analysed frame of the infant's contact with the object display. An α angle value from 90 to 180° indicates that the infant is engaged in a one-handed grasping action. Full size image To assess infants' grasping ability, we measured one-handed grasping in a modified version of the grasping task [32] . In the grasping task, we measured whether infants were able to perform one-handed grasping and the angle, α, as an index of one-handed grasping ability (Methods and Fig. 2b ). Grasping ability of each infant age group Most 4-month-old infants (11/12) were unable to perform either one-handed or two-handed grasping, in that observed α values fell outside limits of acceptable grasping angles. By contrast, a large majority of the 6-, 8-, 10-month-old infants (11 of 12 in each age group) could perform one-handed grasping on more than three of eight trials, whereas only one of the twelve 4-month-olds could ( P <0.001, Fisher's exact test, two-tailed). Thus, there was a significant improvement in grasping ability between 4 and 6 months. On the other hand, with regard to values of the angle α, one-way analysis of variance (ANOVA) with 'Age' (6, 8, and 10 months) as a between-participants factor revealed that differences among the older infants, aged 6-, 8-, and 10-months, were significant ( F 2, 30 =9.472, P =0.001). Post hoc testing (Bonferroni) showed significant differences between 6-month-olds and 10-month-olds ( P <0.001 for 6–10 contrast), and between 8-month-olds and 10-month-olds ( P =0.039 for 8–10 contrast); however, no differences emerged between 6-month-olds and 8–month-olds ( P =0.310 for 6–8 contrast). Together, these analyses indicate that grasping ability continues to develop with age even if infants can grasp an object ( Fig. 3 ). 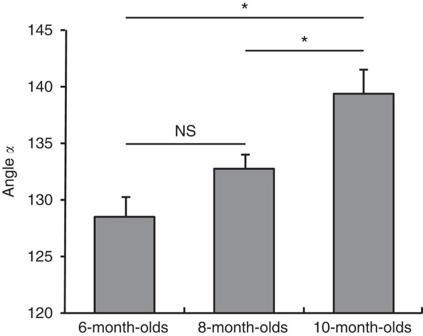Figure 3: Mean angle α as a function of age for older infants. Older infants were 6 (n=11), 8 (n=11), and 10-month-olds (n=11). Asterisks indicate statistical significance,P<0.05; NS, not significant. Error bars are s.e.m. Figure 3: Mean angle α as a function of age for older infants. Older infants were 6 ( n =11), 8 ( n =11), and 10-month-olds ( n =11). Asterisks indicate statistical significance, P <0.05; NS, not significant. Error bars are s.e.m. Full size image Action prediction ability of each age group We compared gaze behaviour across age and condition ( Fig. 4 ), using a repeated-measures ANOVA with 'Action' (GH, BH, MC) as a within-participants factor and 'Age' (4, 6, 8, and 10 months, and adult) as a between-participants factor. The ANOVA revealed significant main effects of Action ( F 2, 110 =31.147, P <0.001) and Age ( F 4, 55 =50.664, P <0.001), and a significant interaction ( F 8, 110 =5.422, P <0.001). Separate ANOVAs were then carried out for each age group. For 4-month-olds, who could not reliably grasp, we found no difference in the time of gaze arrival at the goal between conditions ( F 2, 22 =0.462, P =0.636). In contrast, we found significant between-condition differences for the 6-, 8-, 10-month-olds, and adults (all ages, all F 2, 22 >9.409, P <0.002). Post hoc testing (Bonferroni) revealed that 6-, 8-, and 10-month-olds exhibited significantly more predictive eye movements in the GH condition than in other conditions (across all ages, all P <0.034 for GH-BH contrasts, all P <0.004 for GH-MC, and all P >0.238 for BH-MC). Adults had a different pattern, showing significantly more predictive eye movements in the GH and MC conditions than in the BH condition (GH-BH, P =0.004; GH-MC, P =1.000; BH-MC, P =0.042). 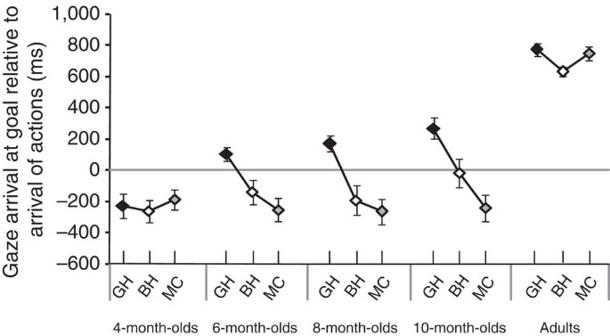Figure 4: Time of gaze arrival at the goal relative to arrival time of each agent's action for each age group. The time of agent's actions in each condition/age group is represented by a horizontal line at 0 ms. Positive relative times of the arrival of gaze at the goal area indicate that gaze precedes the agent's arrival (predictive); negative values indicate gaze arrival after agent arrival (non-predictive). Each age group isn=12. Error bars are s.e.m. Figure 4: Time of gaze arrival at the goal relative to arrival time of each agent's action for each age group. The time of agent's actions in each condition/age group is represented by a horizontal line at 0 ms. Positive relative times of the arrival of gaze at the goal area indicate that gaze precedes the agent's arrival (predictive); negative values indicate gaze arrival after agent arrival (non-predictive). Each age group is n =12. Error bars are s.e.m. Full size image Other follow-up ANOVAs focused upon age differences. Significant effects of Age emerged in all three Action conditions (all F 4, 55 >21.716, P <0.001). Post hoc testing (Bonferroni) was conducted in each condition. In GH condition, there were significant differences between 4-month-olds and older age groups (all P <0.02 for 4–6, 4–8, 4–10, and 4-adults contrasts) and between infants 6 months and older and adults (all P <0.01 for 6-adults, 8-adults, and 10-adults contrasts) but not among 6-, 8-, and 10-month old infants (all P >0.543 for 6–8, 6–10, and 8–10 contrasts). In BH condition, there are significant differences between each infant age group and adults (all P <0.001 for 4-adults, 6-adults, 8-adults, and 10-adults contrasts) but not between 4-, 6-, 8-, and 10-month old infants (all P >0.286 for 4–6, 4–8, 4–10, 6–8, 6–10, and 8–10 contrasts). In MC condition, significant differences appeared between each infant age group and adults (all P <0.001 for 4-adults, 6-adults, 8-adults, and 10-adults contrasts) but not among 4-, 6-, 8-, and 10-month old infants (all P =1.000 for 4–6, 4–8, 4–10, 6–8, 6–10, and 8–10 contrasts). These findings indicate that the oculomotor skills to track the objects do not differ among infants of these age groups in BH and MC conditions. Importantly, infants 6 months and older shifted their gaze to the action goal before the hand arrived in the GH condition; for these ages, the difference between gaze arrival and action (zero) reflected significant anticipation of the goal (for all older ages, t 11 >2.383, all P <0.037, one-sample t -test, two-tailed). By contrast, for these same age groups, gaze arrival in the BH condition did not differ significantly from zero (all t 11 <2.060, all P >0.063). Finally, in the MC condition, gaze lagged the goal for all these infant age groups and these differences were statistically significant (all ages, all t 11 >2.852, all P <0.017). In contrast, to these analyses, the 4-month-olds shifted their gaze to the action goal only after the agent arrived; that is, they showed significant lagging in all three Action conditions (all conditions, all t 11 >2.909, P <0.015). By contrast, adults shifted their gaze to the action goal before the agent arrived in all conditions (all conditions, all t 11 >17.481, all P <0.001). The relation between action prediction and motor ability Finally, to further assess developmental correspondence we conducted a correlation analysis between gaze behaviour and grasping ability in infants 4 months and older, analysing all data within ±2 s.d. of the mean (GH condition, n =31; BH condition, n =31; MC condition, n =32). Grasping ability was significantly related to eye movements in the GH and BH conditions, but not in the MC condition (GH, r =0.44, P =0.014; BH, r =0.44, P =0.014; MC, r =0.09, P =0.636). After controlling for age, partial correlations revealed that this significant relationship was only present in the GH condition (GH, r =0.41, P =0.026; BH, r =0.29, P =0.126; MC, r =0.11, P =0.567; Fig. 5 ). 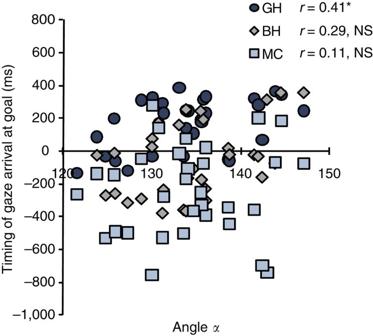Figure 5: Scatter plots showing the relationship between action prediction and grasping ability in infants. Dark blue circles, grey diamonds, and light blue squares represent the correlational relationships, respectively, between grasping ability and gaze arrival time at the goal for three action conditions: grasping hand (GH,n=31), back of hand (BH,n=31), and mechanical claw (MC,n=32). Pearson'srreflects the partial correlation between timing of gaze arrival at the goal and grasping ability in each condition after controlling for age. Asterisk indicates statistical significance,P<0.05; NS, not significant. Figure 5: Scatter plots showing the relationship between action prediction and grasping ability in infants. Dark blue circles, grey diamonds, and light blue squares represent the correlational relationships, respectively, between grasping ability and gaze arrival time at the goal for three action conditions: grasping hand (GH, n =31), back of hand (BH, n =31), and mechanical claw (MC, n =32). Pearson's r reflects the partial correlation between timing of gaze arrival at the goal and grasping ability in each condition after controlling for age. Asterisk indicates statistical significance, P <0.05; NS, not significant. Full size image This study demonstrates that the ability to predict the action goals of others emerges in infancy as early as six months and this emergence co-occurs with the onset of infants' own motor ability of same action. There is also a correspondence relationship between action prediction ability and motor ability of same action. For this task, the ability to predict a motor action becomes evident at six months, which is a younger age than has been demonstrated in a previous study [22] . This indicates that infants can predict action goals of others only when the observed actions of others are within a repertory of actions that the infants themselves can perform. Also, the fact that 4-month-olds are less capable in anticipating an action goal than older infants is not due a general inability of 4-month-olds to predict future events with their gaze, because 4-month-olds can predict the reappearance of temporarily occluded objects with their gaze [38] , [39] . Moreover, we found no significant age differences among 4-, 6-, 8-, and 10-month old infants in gazes of BH and MC conditions, indicating that the actual capacity to track objects does not differ among infants of all age groups. Also, the correlation we observed for the GH condition cannot be explained by general development, because this correlation was significant even with age partialled out. Thus, our results suggest a developmental correspondence between predicting others' action goals and manifesting those same actions during early infancy. Importantly, infants 6 months and older were able to make goal-related predictions for goal-directed actions performed by humans (GH condition) but not for non-goal-directed actions performed by humans (BH condition) or goal-directed actions made by an inanimate agent (MC condition). This pattern of results cannot be explained by the possibility that the motion itself created by a moving hand (or claw) elicits proactive eye movements regardless of actor type or goal direction. Likewise, the findings exclude the possibility that results were due to differences in visual properties between the different agents' actions. The visual properties of the action video in the GH and BH conditions were very similar. However, infants predicted the action goal only in GH condition, but not in either the BH or the MC condition. Thus, the findings show that infants 6 months and older are able to selectively predict the goal of humans' goal-directed actions. This finding not only confirms the results of recent neurophysiological studies demonstrating MNS function in 6-month-old infants [14] , [15] , but is also consistent with studies of 9-month-olds showing that motor activation occurs during the observation of goal-directed actions, but not non-goal-directed actions [18] . Altogether, our findings support the MNS account of understanding action through a direct matching process [12] , [13] . Interestingly, we found different patterns of gaze behaviour for adults compared with infants 6 months and older. Adults made goal-related predictions about the inanimate agent's goal-directed actions to the same extent as for a human actor. In contrast, infants 6 months and older could not predict the inanimate agent's action as quickly as for the human actor. These different gaze patterns indicate different developmental trajectories for the ability to predict human goal-directed actions and an inanimate agent's goal-directed movements. We propose two possibilities to account for this discrepancy in prediction ability between adults and infants. First, it is likely that adults are able to predict the action goals by simulating the inanimate agent's actions even if they do not correspond to their own motor representations. It was recently proposed that the MNS is flexible and modulated by experience [40] , [41] , [42] . In accord with this proposal, a recent behavioural study reported that sensorimotor experience configures responses of the MNS to the actions of inanimate agents [43] . Furthermore, one functional magnetic resonance imaging (fMRI) study has demonstrated that both human and inanimate agent's actions strongly activated cortical structures of the MNS [44] . Second, adults may predict the inanimate agent's action goals by referring to representations of tool-use actions. Recent electrophysiological evidence in monkeys suggested that mirror neurons responded to the observation of tool-use actions after visual exposure to these actions [45] or motor training [46] . In addition, recent neurophysiological evidence in human adults suggests that the primary motor cortex is activated during the observation of tool-use actions and that this activation is modulated by the observer's experience of performing that action [47] . With any of these possibilities, as experience is acquired during development, infants would be expected to become more able to predict an inanimate agent's action goals. Moreover, the ability to predict goal-directed actions performed by humans, which is directly linked to infants' own motor ability, may generalize with appropriate experience to the goal-directed actions of inanimate agents. In conclusion, our findings show a developmental correspondence between action understanding and motor ability to perform that same action in early infancy, indicating that the ability to predict others' action goals requires the ability to perform the corresponding motor action. This finding provides direct ontogenetic evidence to converge on the claim inherent in the MNS hypothesis that goal prediction involves a direct matching process. Determining when and how the ability to predict the action goals of inanimate objects emerges in ontogeny will require further research. Participants Infant participants were full term, with 6 female and 6 male at each of the following age levels: 4-months (mean=4 mo 14 days; range, 4 mo 1 day to 4 mo 27 days); 6-months (mean=6 mo 14 days; range, 6 mo 2 days to 6 mo 27 days); 8-months (mean=8 mo 17 days; range, 8 mo 3 days to 8 mo 27 days) and 10-months (mean=10 mo 11 days; range, 10 mo 1 day to 10 mo 27 days). Twelve right-handed, healthy adults (6 female, 6 male; mean age=21.4 years; range, 18 years to 24 years) also participated. Twenty additional infants and two additional adults were tested but excluded from the analyses because of inattentiveness (18 infants and two adults who completed less than two trials of each condition), parental interference (one) or technical errors (one). The parents of the infants, and the adult participants, provided written informed consent. The experiments were approved by the ethics review board at the Department of Psychology, Kyoto University. Apparatus and displays A Tobii T60 Eye Tracker (Tobii Technology) was used to record participants' gaze movements. An integrated 17′′ TFT monitor presented the movie stimuli using Tobii Studio (Tobii Technology). Adult participants were seated on a chair and infants were seated on the lap of a parent, with eyes approximately 60 cm from the monitor. A five-point calibration was administered before recording. The grasping task involved one object display consisting of a single attractive ball (8.5×6.0×6.0 cm) attached with Velcro to the centre of a transparent plastic plate (30×45 cm, 0.3 cm thick). Small rings were affixed with Velcro to the opposite side of the plate to which the ball was attached to attract the infants' attention. A video camera attached to the ceiling of the experimental room recorded the actions from a bird's eye view. Stimuli and procedure Participants were presented with three types of videos (subtending 19.9°×16.1° of the visual angle) where agents reached towards one of two toys placed at the upper part of the screen from the participant's perspective. The types of videos were 'grasping hand' in the GH condition, 'back of hand' in the BH condition, and 'mechanical claw' in the MC condition ( Fig. 1 ). Each video consisted of five components. The hand/claw was out of the frame for the first 3 s of the video ( Fig. 1a ). The hand (or claw) then appeared from the bottom of the frame and moved upward (2 s), stopped in the lower part of the scene (1 s; Fig. 1b ), moved towards one of the two toys (2 s), and stopped at the target toy (1 s; Fig. 1c ). The hand or claw in the GH and MC conditions grasped the target toy, whereas the agents in the BH condition placed the back of the hand on the target toy. The videos had a total duration of 9 s and were edited using Adobe Premiere 6.5 (Adobe Systems Inc.) to control the duration of each component. There were six trials in each of the three conditions. The video stimuli in each of the three conditions contained a unique pair of objects. Attractive animations with sound were inserted between each trial to keep infants' attention focused on the monitor. The three possible presentation orders of the three conditions were counterbalanced across participants (for example, GH–BH–MC, BH–MC–GH, MC–GH–BH). The direction of the agent's action (that is, towards one or the other object) was counterbalanced in an ABBABA order (GH condition), an ABABBA order (BH condition), or an AABABB order (MC condition). The direction of the agent's first action in each condition was controlled such that it was not successive across conditions (for example, Left (L) –Right (R) –L, R–L–R). After recording of eye movements while they viewed the videos, infants completed a modified version of the grasping task [32] . In the grasping task, infants were seated on the lap of a parent and presented with an object display. The experimenter held the display in front of them, then moved it out of the infant's reach ( ∼ 1.5 m away) and shook it until the infant attended to the object. After confirming the infant's attention, the experimenter slowly brought the object display to a position almost within reach. The presentation of the object display ended when the infant touched, grasped or detached the object from the plastic plate. If the infant showed no attempt to reach towards the object, the object display was first shaken and then removed from within reach of the infant after 60 s. Infants experienced a total of eight object presentations. Data analyses All gaze data were analysed using Tobii's standard statistics package (Tobii Technology). We defined three areas of interest (AOI; Fig. 2a ): one covering the target object ('goal AOI'); one covering the position where agents stopped before starting to move towards the target object ('agent AOI'); and one covering the trajectory of the agent's movement ('trajectory AOI'). Data were included in the analyses only if the participants fulfilled the following three criteria for at least two trials of each condition. Participants had to fixate on both the objects and the agent, before the agent moved to the target object, and then fixated on the agent AOI for 200 ms [22] after the agent had moved or fixated on the agent in the trajectory AOI for 200–600 ms while the agent was moving to the target object, and finally fixated on the goal AOI before the video ended. The first trial of each condition was excluded from analysis because the gaze shift of the first trial is not predictive [22] . Some adults and many of the infants exhibited occasional gaze shifts to the objects before the agents had started to move to the target objects. This gaze behaviour did not constitute predictive eye movement but merely indicated that the participant associated the agent with the object. However, in these cases, the participants shifted their gaze back to the agents as the agents moved towards the target objects. Thus, we applied wide criteria for the starting point of the gaze shift, after the agent had moved for 200 ms or while the agent was moving to the target object for 200–600 ms. The timing of the gaze shift to the goal AOI was compared with the arrival of the agent's action. The arrival of the agent's action was defined as the time when half of the hand (in the GH and BH conditions) or claw (in the MC condition) was located within the goal AOI. If the participant's gaze arrived at the goal AOI before the agent, the trial was regarded as predictive (positive score). In contrast, if the participant's gaze arrived at the goal AOI after the agent arrived at the goal AOI, the trial was not regarded as predictive (negative score). For the grasping task, the time of the video frame at the moment when the infant's hand contacted the object was analysed. Trials for which the infant performed a bimanual grasping action were excluded from the analyses. Infants were required to show a one-handed grasping action (left- or right-handed action) in at least three of the eight trials to be included in the analyses. If infants did a one-handed grasping action in more than three of the eight trials, we regarded the infants as being able to grasp. Grasping ability was measured in terms of the angle, α, as shown in Figure 2b . The angle α is an index of the development of the one-handed grasping action [32] and was calculated by measuring the angle of a straight line defined by the infant's two hands (the apex of the junction of the thumb and index finger) when crossed by an imaginary line projecting frontally from the infant ( Fig. 2b ). If infants grasped for the objects with their left hand, we reversed the red right-angled triangle from one side to the other side and calculated the angle α in the same way. The angle α value of 90° corresponded to a perfect alignment of the hands in a two-handed reach. Therefore, the angle α value deviates from 90° towards 180°, and bigger angle α value indicates more mature one-handed grasping. If the angle α was over 90°, the infant was considered to be engaged in a one-handed grasping action. The angle was measured with Adobe Photoshop Elements 5.0 (Adobe Systems Inc.) from the video frame. How to cite this article : Kanakogi, Y. and Itakura, S. Developmental correspondence between action prediction and motor ability in early infancy. Nat. Commun. 2:341 doi: 10.1038/ncomms1342 (2011).